An acetylation switch controls TDP-43 function and aggregation propensity TDP-43 pathology is a disease hallmark that characterizes amyotrophic lateral sclerosis (ALS) and frontotemporal lobar degeneration (FTLD-TDP). Although a critical role for TDP-43 as an RNA-binding protein has emerged, the regulation of TDP-43 function is poorly understood. Here, we identify lysine acetylation as a novel post-translational modification controlling TDP-43 function and aggregation. We provide evidence that TDP-43 acetylation impairs RNA binding and promotes accumulation of insoluble, hyper-phosphorylated TDP-43 species that largely resemble pathological inclusions in ALS and FTLD-TDP. Moreover, biochemical and cell-based assays identify oxidative stress as a signalling cue that promotes acetylated TDP-43 aggregates that are readily engaged by the cellular defense machinery. Importantly, acetylated TDP-43 lesions are found in ALS patient spinal cord, indicating that aberrant TDP-43 acetylation and loss of RNA binding are linked to TDP-43 proteinopathy. Thus, modulating TDP-43 acetylation represents a plausible strategy to fine-tune TDP-43 activity, which could provide new therapeutic avenues for TDP-43 proteinopathies. TDP-43 is a highly conserved and ubiquitously expressed nuclear protein that contains two RNA-recognition motifs (RRMs) involved in RNA and DNA binding, as well as a glycine-rich C-terminal sequence, which harbours the majority of the ALS-linked mutations [1] , [2] . TDP-43 has diverse cellular roles in regulating RNA splicing and RNA stability as well as other gene regulatory functions [3] , [4] , [5] . High-throughput sequencing approaches have shown that TDP-43 binds ~6,000 genes and regulates target RNAs that are essential for proper neuronal development and synaptic function [4] , [5] , [6] . In addition to RNA targets, TDP-43 binds to proximal gene promoters and regulates gene expression of SP-10 (acrosomal vesicle protein 1) and cdk6 (cyclin-dependent kinase 6) [7] , [8] , [9] , suggesting a distinct role in gene transcription. Studies have also implicated TDP-43 as a stress-responsive RNA-associated factor required for local translation in the cytoplasm [10] . Supporting this finding, TDP-43 is a major component of neuronal RNA granules and cytoplasmic stress granules (SGs) [11] , [12] , [13] , [14] , which are active sites of RNA regulation and sorting during exposure to stress. Thus, the normal physiological functions of TDP-43 could involve the response to environmental stress via regulation of downstream genes and RNAs. Although the identification of TDP-43 target RNAs has been a major focus recently, the mechanisms that regulate TDP-43 function remain poorly understood. TDP-43 is predominantly nuclear localized; however, pathological TDP-43 found in the diseased brain and spinal cord becomes abnormally aggregated primarily in the cytoplasm, which has been linked to onset and/or progression of TDP-43 proteinopathy by several pathogenic mechanisms [15] , [16] . The physical presence of cytoplasmic aggregates could exert a toxic gain of function via impaired vesicle trafficking as well as cytoskeletal abnormalities [17] , [18] . In addition, substantial evidence indicates that TDP-43 aggregates induce loss of normal nuclear TDP-43 functions, as nuclear depletion of normally soluble TDP-43 due to TDP-43 aggregates led to loss of splicing and transcription activities in cultured cells and transgenic mice [19] , [20] , [21] , [22] , [23] . Pathological TDP-43 is abnormally phosphorylated on C-terminal serine residues (Ser-403/404 and Ser-409/410) by multiple kinases [24] , [25] , [26] , [27] and has emerged as a disease-specific marker of human TDP-43 proteinopathy [16] , [25] , [28] . Although phospho-TDP-43 immunoreactivity is valuable as a postmortem diagnostic tool, the significance of phosphorylation as it relates to TDP-43 biology is not clear. Indeed, several studies have indicated that phosphorylation actually prevents rather than promotes TDP-43 aggregation [29] , [30] , suggesting that additional signalling mechanisms likely exist to modulate TDP-43 functions and aggregate formation in diseased individuals. Lysine acetylation has emerged as a major covalent modification controlling diverse cellular processes and has been implicated in Alzheimer’s disease (AD) and other neurodegenerative disorders [31] , [32] , [33] , [34] , [35] . For example, we demonstrated that acetylation of misfolded tau proteins marks mature neurofibrillary tangles (NFTs) in AD and related tauopathies and represents a disease-specific marker of AD pathology [31] , [33] , [34] . In addition to tau, a global proteomics approach identified ~1,750 proteins that are subject to lysine acetylation, including a distinct subset of RNA-binding proteins and associated factors [36] . As TDP-43 is an RNA-binding protein implicated in ALS, we asked whether TDP-43 is subject to acetylation, a modification that could regulate cellular processes linked to ALS pathogenesis. Here, we show that acetylation occurs on TDP-43 lysine residues within the RNA-binding domains (RRMs), which functionally abrogates RNA binding and promotes the accumulation of insoluble TDP-43 aggregates. Our identification of acetylated TDP-43 lesions present in ALS patient spinal cord highlights a novel pathological signature and provides a rationale to explore TDP-43 acetylation as a potential therapeutic target in ALS and related TDP-43 proteinopathies. TDP-43 is subject to acetylation at specific lysine residues To determine whether TDP-43 is acetylated, co-transfection experiments were performed with TDP-43 and the acetyltransferase Creb-binding protein (CBP), followed by immunoprecipitation and immunoblotting using a pan-acetyl-lysine antibody. Ectopically expressed myc-tagged wild-type (WT) TDP-43 was prominently acetylated only in the presence of CBP ( Fig. 1a and Supplementary Fig. 1 ). To further confirm TDP-43 acetylation, WT TDP-43 expressing cells were incubated with [ 3 H]-acetate, and we observed the incorporation of [ 3 H]-labeled acetyl groups onto TDP-43 by SDS–polyacrylamide gel electrophoresis (SDS–PAGE) and autoradiography ( Fig. 1b and Supplementary Fig. 1 ). Interestingly, mutating the TDP-43 nuclear localization sequence (TDP-43-ΔNLS) led to increased TDP-43 acetylation on mislocalization to the cytoplasm ( Fig. 1c and Supplementary Fig. 1 ), a compartment where TDP-43 forms inclusions in the diseased human brain and spinal cord. Although CBP is predominantly nuclear localized, immunofluorescence analysis indicated that a subpopulation of transfected CBP was recruited to cytoplasmic TDP-43-ΔNLS foci ( Fig. 1d ), thereby implicating direct CBP-mediated acetylation of TDP-43. There were no appreciable differences in acetylation among a panel of ALS-associated TARDBP mutations also directed to the cytoplasm ( Supplementary Fig. 2 ), consistent with the mild aggregation phenotype observed for these mutations in cultured cell lines [2] . 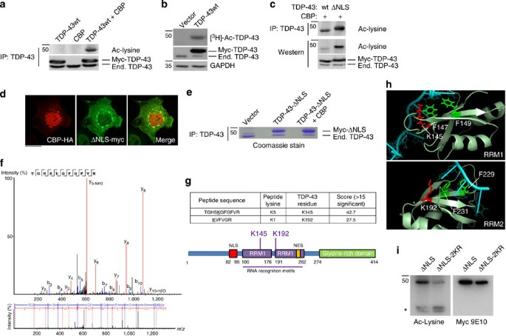Figure 1: TDP-43 is subject to lysine acetylation within the RNA-binding domain. (a) QBI-293 cells were transfected with TDP-43 in the presence or absence of the acetyltransferase CBP and acetylated TDP-43 was evaluated by immunoprecipitation (anti-TDP-43 clone 171) followed by immunoblotting using an anti-acetylated lysine antibody. (b) Cells transfected with wild-type TDP-43 were pulse-labelled with [3H]-acetate for 2 h followed by immunoprecipitation and analysis by SDS–PAGE and autoradiography for 2 weeks. Total cellular lysates representing 5% total input were immunoblotted using anti-TDP-43 and GAPDH antibodies. (c) TDP-43 acetylation assay was performed similar to (a) above using either wild-type TDP-43 or the cytoplasmic mutant TDP-43-ΔNLS in the presence of the acetyltransferase CBP. Samples were analysed by immunoprecipitation (top panel) and direct immunoblotting (bottom panels) using acetylated lysine and total TDP-43 antibodies. (d) Double-labelling immunofluorescence was performed on cells transfected with CBP and TDP-43-ΔNLS using anti-HA and anti-myc antibodies, respectively. The merge indicates co-localization of CBP with cytoplasmic-localized TDP-43. Scale bar, 25 μm. (e,f) Cells were transfected with vector alone or TDP-43-ΔNLS in the absence or presence of CBP and total TDP-43 was immunoprecipitated, separated by SDS–PAGE followed by gel excision, and analysed by mass spectrometry, which identified the K145-acetylated peptide shown inf. (g) CBP-mediated acetylation of two lysine residues clustered within the RNA-binding regions with significant ion scores andP-values are shown. (h) Crystal structure analysis of RNA-binding domains RRM1 and RRM2 bound to DNA (Protein Data Bank entries 3D2W and 4IUF) illustrates Lys-145 and Lys-192 (shown in red) adjacent to critical Phe residues (shown in green) in the context of bound DNA (shown in cyan). (i) Cytoplasmic TDP-43-ΔNLS or a comparable construct containing K→R mutations at Lys-145 and Lys-192 (TDP-43-ΔNLS-2KR) were analysed by immunoblotting in the presence of CBP and HDAC inhibitors (nicotinamide/TSA) to promote full TDP-43 acetylation. The asterisk (*) indicates acetylated cross-reactive bands that are unaltered by TDP-43. Figure 1: TDP-43 is subject to lysine acetylation within the RNA-binding domain. ( a ) QBI-293 cells were transfected with TDP-43 in the presence or absence of the acetyltransferase CBP and acetylated TDP-43 was evaluated by immunoprecipitation (anti-TDP-43 clone 171) followed by immunoblotting using an anti-acetylated lysine antibody. ( b ) Cells transfected with wild-type TDP-43 were pulse-labelled with [ 3 H]-acetate for 2 h followed by immunoprecipitation and analysis by SDS–PAGE and autoradiography for 2 weeks. Total cellular lysates representing 5% total input were immunoblotted using anti-TDP-43 and GAPDH antibodies. ( c ) TDP-43 acetylation assay was performed similar to ( a ) above using either wild-type TDP-43 or the cytoplasmic mutant TDP-43-ΔNLS in the presence of the acetyltransferase CBP. Samples were analysed by immunoprecipitation (top panel) and direct immunoblotting (bottom panels) using acetylated lysine and total TDP-43 antibodies. ( d ) Double-labelling immunofluorescence was performed on cells transfected with CBP and TDP-43-ΔNLS using anti-HA and anti-myc antibodies, respectively. The merge indicates co-localization of CBP with cytoplasmic-localized TDP-43. Scale bar, 25 μm. ( e , f ) Cells were transfected with vector alone or TDP-43-ΔNLS in the absence or presence of CBP and total TDP-43 was immunoprecipitated, separated by SDS–PAGE followed by gel excision, and analysed by mass spectrometry, which identified the K145-acetylated peptide shown in f . ( g ) CBP-mediated acetylation of two lysine residues clustered within the RNA-binding regions with significant ion scores and P -values are shown. ( h ) Crystal structure analysis of RNA-binding domains RRM1 and RRM2 bound to DNA (Protein Data Bank entries 3D2W and 4IUF) illustrates Lys-145 and Lys-192 (shown in red) adjacent to critical Phe residues (shown in green) in the context of bound DNA (shown in cyan). ( i ) Cytoplasmic TDP-43-ΔNLS or a comparable construct containing K→R mutations at Lys-145 and Lys-192 (TDP-43-ΔNLS-2KR) were analysed by immunoblotting in the presence of CBP and HDAC inhibitors (nicotinamide/TSA) to promote full TDP-43 acetylation. The asterisk (*) indicates acetylated cross-reactive bands that are unaltered by TDP-43. Full size image To identify putative lysine acetylation sites, TDP-43-ΔNLS was co-transfected with CBP and subsequently immunoprecipitated from cell lysates using a TDP-43-specific monoclonal antibody (clone 171), resulting in enrichment of TDP-43-ΔNLS that was readily detected by standard SDS–PAGE and Coomassie stained gels ( Fig. 1e and Supplementary Fig. 3 ). TDP-43 protein bands were gel excised, trypsin digested and analysed by mass spectrometry using nanoLC/nanospray/MS/MS. On the basis of ~75% sequence coverage of human TDP-43, we identified two major acetylated sites in the RNA-binding domains ( Fig. 1f and Supplementary Fig. 4 ); Lys-145 in RRM1, which spans residues 105–169, and Lys-192 immediately adjacent to RRM2, which spans residues 194–257 (see Fig. 1g for schematic of TDP-43 acetylation sites). Amino-acid mapping onto known crystal structures of either RRM1 or RRM2 bound to target DNA [37] , [38] showed that acetylation of the Lys-145 and Lys-192 side chains could potentially interact with and alter nucleic acid binding ( Fig. 1h , Lys residues highlighted in red). Supporting this possibility, both lysines are adjacent to neighbouring Phe residues in RRM1 (Phe-147/149) and RRM2 (Phe-229/231), previously shown to interact directly with nucleic acids [39] ( Fig. 1h , Phe residues highlighted in green). To determine whether Lys-145 and Lys-192 represent major acetylated residues in TDP-43, we generated a TDP-43-ΔNLS mutant containing lysine substitutions (TDP-43-ΔNLS-2KR). The acetylation-deficient mutant showed reduced but not completely abrogated acetylation ( Fig. 1i and Supplementary Fig. 5 ), suggesting Lys-145 and Lys-192 are dominant sites of acetylation, although additional acetylated lysines may be present that are not detectable using this approach. TDP-43 acetylation enhances aggregate formation To determine the consequences of TDP-43 acetylation at these lysine residues, acetylation mimic (K→Q) and non-mimic (K→R) mutants were generated and analysed by immunofluorescence microscopy. As shown in Fig. 2a , nuclear WT TDP-43 exhibits a diffuse nucleoplasmic pattern with punctate nuclear bodies as previously reported [23] , [40] . However, a single acetylation mimic TDP-K145Q, and, more prominently, the double acetylation mimic TDP-2KQ displayed a severely stippled nuclear localization in ~65% of cells (see Fig. 2b for quantification), which closely resembled the TDP-4FL RNA-binding-deficient Phe mutant [41] , strongly suggesting impaired RNA binding. Strikingly, targeting acetylation to the cytoplasm using TDP-43-ΔNLS containing single or double acetylation mimics showed a distinct phenotype characterized by cytoplasmic inclusions that resembled pathological inclusions seen in ALS and other TDP-43 proteinopathies [16] , [28] , [42] ( Fig. 2a,b , ~75% aggregates for TDP-43-ΔNLS-2KQ). 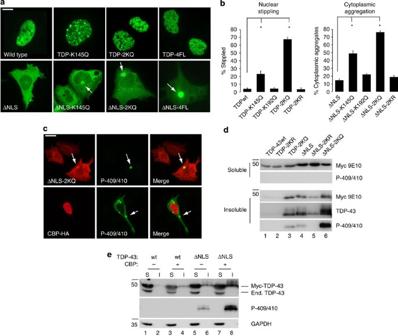Figure 2: TDP-43 acetylation promotes pathological features associated with TDP-43 proteinopathies. (a) Double-labelling immunofluorescence was performed on cells transfected with myc-tagged wild-type TDP-43 or cytoplasmic localized TDP-43-ΔNLS containing the single acetylation mimic (K145Q), double mimic (TDP-2KQ) or 4FL RNA-binding-deficient mutations (F147/149/229/231L). White arrows highlight cytoplasmic accumulation of TDP-43 aggregates. Scale bar, 10 μm. (b) Nuclear stippling and cytoplasmic aggregation phenotypes were quantified for all TDP-43 acetylation-mimic and non-mimic mutants at residues Lys-145 and Lys- 192. Error bars indicate s.e.m., and the single asterisk indicates statistical significance withP-value <0.05 as measured by two-tailed unpairedt-test with unequal variance fromN=3 biological replicates. (c) Cells expressing acetylation-mimic TDP-43-ΔNLS (TDP-43-ΔNLS-2KQ) or CBP-acetylated TDP-43-ΔNLS were analysed by immunofluorescence microscopy using a phospho-TDP-43 antibody (P-409/410) to mark pathological TDP-43 aggregates. Scale bar, 25 μm. (d,e) Soluble (S) and insoluble (I) fractions from cells expressing acetylation-mimics as well as CBP-mediated acetylated TDP-43 were analysed by immunoblotting using the indicated myc-9E10, TDP-43 (1038), phospho-TDP-43 (P409/410) or GAPDH antibodies. Figure 2: TDP-43 acetylation promotes pathological features associated with TDP-43 proteinopathies. ( a ) Double-labelling immunofluorescence was performed on cells transfected with myc-tagged wild-type TDP-43 or cytoplasmic localized TDP-43-ΔNLS containing the single acetylation mimic (K145Q), double mimic (TDP-2KQ) or 4FL RNA-binding-deficient mutations (F147/149/229/231L). White arrows highlight cytoplasmic accumulation of TDP-43 aggregates. Scale bar, 10 μm. ( b ) Nuclear stippling and cytoplasmic aggregation phenotypes were quantified for all TDP-43 acetylation-mimic and non-mimic mutants at residues Lys-145 and Lys- 192. Error bars indicate s.e.m., and the single asterisk indicates statistical significance with P -value <0.05 as measured by two-tailed unpaired t -test with unequal variance from N =3 biological replicates. ( c ) Cells expressing acetylation-mimic TDP-43-ΔNLS (TDP-43-ΔNLS-2KQ) or CBP-acetylated TDP-43-ΔNLS were analysed by immunofluorescence microscopy using a phospho-TDP-43 antibody (P-409/410) to mark pathological TDP-43 aggregates. Scale bar, 25 μm. ( d , e ) Soluble (S) and insoluble (I) fractions from cells expressing acetylation-mimics as well as CBP-mediated acetylated TDP-43 were analysed by immunoblotting using the indicated myc-9E10, TDP-43 (1038), phospho-TDP-43 (P409/410) or GAPDH antibodies. Full size image Acetylation of cytoplasmic TDP-43 using either acetylation-mimic mutations or co-transfected CBP led to the formation of bona fide TDP-43 aggregates that are phosphorylated at Ser-409 and Ser-410 (P-409/410), a disease hallmark of TDP-43 pathology [28] , [43] ( Fig. 2c ). Similarly, solubility assays confirmed that targeting TDP-43 acetylation mimics to the cytoplasm increased P-409/410 levels in insoluble fractions ( Fig. 2d , lane 6 and Supplementary Fig. 6 ). Importantly, acetylation-induced aggregation was not observed with non-mimic K→R substitutions ( Fig. 2d , compare lanes 4–6). Indeed, we attribute the TDP-43 insolubility to acetylation, as co-transfection of CBP similarly enhanced the phosphorylation of TDP-43-ΔNLS that was recovered in the insoluble fraction ( Fig. 2e , lanes 6 and 8 and Supplementary Fig. 6 ). Cytoplasmic TDP-43 acetylation similarly induced aggregation in differentiated Neuro2A cells precluding any cell-type-specific differences in TDP-43 aggregation propensity ( Supplementary Fig. 7 ). Thus, these results support lysine acetylation as a critical determinant of TDP-43 aggregate formation and highlight distinct aggregation pathologies resulting from TDP-43 subcellular localization. Acetylation-mimics impair TDP-43 RNA-regulatory functions Given that the acetylated lysines are located within the RRM domains, we sought to determine whether TDP-43 acetylation functionally altered RNA binding. Recombinant full-length TDP-43 proteins containing acetylation mimic and non-mimic mutations were sequentially extracted from bacteria yielding highly pure TDP-43 proteins by Coomassie staining ( Fig. 3a and Supplementary Fig. 8 ). Consistent with high affinity nucleic acid binding, absorbance readings (A260/280) of WT and TDP-2KR protein preparations indicated the presence of co-purifying nucleic acids that were not abundant in preparations of the TDP-2KQ acetylation-mimic, suggesting a conformational change induced by charge neutralization (that is, Lys → Gln substitutions) that abrogated binding to nucleic acids. To assess the functional consequence of reduced RNA binding to TDP-43, we utilized a cell-based nuclear CFTR splicing assay in which TDP-43 expression facilitates exon 9 skipping of a CFTR minigene ( Fig. 3b and Supplementary Fig. 8 ) [39] , [44] , [45] . As expected, TDP-43 shRNA led to the accumulation of the exon 9 included (unspliced) transcript and a marked reduction in the spliced/unspliced ratio, while WT TDP-43 overexpression reversed this effect by enhancing the exon 9 excluded product ( Fig. 3c ). Consistent with a loss of TDP-43 function, the acetylation-mimic K145Q mutant displayed a partial reduction in the spliced/unspliced ratio relative to the baseline, and a similar but more severe loss of function was observed with the RNA-binding-deficient 4FL mutant, which completely abrogated RNA binding [39] ( Fig. 3c , compare WT with K145Q and 4FL). 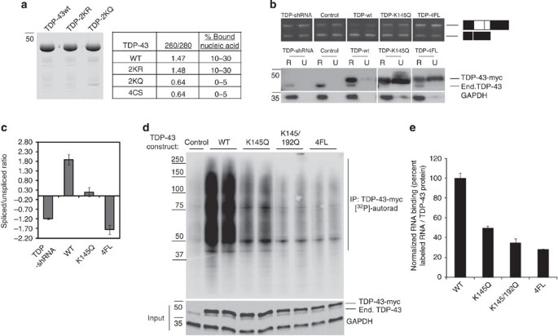Figure 3: TDP-43 acetylation impairs RNA-regulatory functions. (a) Recombinant full-length wild-type TDP-43, non-mimic TDP-2KR and acetylation mimic TDP-2KQ mutants were purified by a sequential extraction according to the methods, and co-purifying nucleic acid was quantified by measuring absorbance at 260/280 nm (A260/280). The percent co-purifying nucleic acid is estimated based on known A260/280 values, which are significantly reduced for TDP-2KQ and 4CS mutant proteins11, indicating reduced association of these proteins with total extracted nucleic acids. (b) Cells expressing vector control, TDP-43shRNA, wild-type TDP-43, TDP-K145Q or RNA-binding-deficient 4FL plasmids were co-transfected with a CFTR minigene. TDP-43 protein levels were determined by immunoblotting, and spliced/unspliced CFTR transcripts were assessed by RT–PCR using specific primers flanking exon 9. (c) RT–PCR products were quantified using the Agilent 2100 Bioanalyzer and relative values of CFTR transcripts are represented as a log ratio of spliced/unspliced products. All samples are normalized to the vector control. Splicing analysis was performed using three independent experiments (N=3), and error is displayed as s.e.m. (d) Crosslinking immunoprecipitation (CLIP) assay was performed on cells expressing wild-type TDP-43, K145Q, 2KQ (K145/192Q) or TDP-4FL plasmids. TDP-43-bound RNAs were immunoprecipitated using anti-myc (9E10), end-labelled with [32P]-ATP and visualized using bis-tris gel immunoblotting followed by phosphorimaging analysis. Shown is a representative image containing duplicate samples for each construct that was obtained fromN=3 independent experiments. (e) TDP-43-associated RNAs were quantified using TYPHOON software and normalized to total TDP-43 protein inputs, as determined by immunoblotting with an anti-myc antibody shown ind. All mutants analysed (K145Q, K145Q/192Q, 4FL) showed significant reduction in RNA-binding compared with WT as assessed by Student’st-test (P-value ≤0.01) fromN=3 independent experiments. Error bars indicate s.d. of normalized intensity signals derived from experimental replicates. Figure 3: TDP-43 acetylation impairs RNA-regulatory functions. ( a ) Recombinant full-length wild-type TDP-43, non-mimic TDP-2KR and acetylation mimic TDP-2KQ mutants were purified by a sequential extraction according to the methods, and co-purifying nucleic acid was quantified by measuring absorbance at 260/280 nm (A260/280). The percent co-purifying nucleic acid is estimated based on known A260/280 values, which are significantly reduced for TDP-2KQ and 4CS mutant proteins [11] , indicating reduced association of these proteins with total extracted nucleic acids. ( b ) Cells expressing vector control, TDP-43shRNA, wild-type TDP-43, TDP-K145Q or RNA-binding-deficient 4FL plasmids were co-transfected with a CFTR minigene. TDP-43 protein levels were determined by immunoblotting, and spliced/unspliced CFTR transcripts were assessed by RT–PCR using specific primers flanking exon 9. ( c ) RT–PCR products were quantified using the Agilent 2100 Bioanalyzer and relative values of CFTR transcripts are represented as a log ratio of spliced/unspliced products. All samples are normalized to the vector control. Splicing analysis was performed using three independent experiments ( N =3), and error is displayed as s.e.m. ( d ) Crosslinking immunoprecipitation (CLIP) assay was performed on cells expressing wild-type TDP-43, K145Q, 2KQ (K145/192Q) or TDP-4FL plasmids. TDP-43-bound RNAs were immunoprecipitated using anti-myc (9E10), end-labelled with [ 32 P]-ATP and visualized using bis-tris gel immunoblotting followed by phosphorimaging analysis. Shown is a representative image containing duplicate samples for each construct that was obtained from N =3 independent experiments. ( e ) TDP-43-associated RNAs were quantified using TYPHOON software and normalized to total TDP-43 protein inputs, as determined by immunoblotting with an anti-myc antibody shown in d . All mutants analysed (K145Q, K145Q/192Q, 4FL) showed significant reduction in RNA-binding compared with WT as assessed by Student’s t -test ( P -value ≤0.01) from N =3 independent experiments. Error bars indicate s.d. of normalized intensity signals derived from experimental replicates. Full size image Finally, we utilized a crosslinking immunoprecipitation assay (CLIP) [4] , [5] to directly assess the RNA-binding activity of acetylated TDP-43. As expected, WT TDP-43 contains functional RNA-binding properties [5] and physically bound to total cellular RNAs as determined by TDP-43 gel migration as ~50–250 kDa protein/RNA complexes ( Fig. 3d , see TDP-43 bound target RNAs within the bracket, and Supplementary Fig. 8 ). However, a single acetylation-mimic mutant, and more prominently the double mutant (TDP-K145Q or TDP-2KQ), showed an ~50–65% decrease in RNA binding, a partial loss of function that approached that observed with the RNA-binding-deficient 4FL mutant (~ 70% decrease), as determined by quantification and normalization of crosslinked high molecular weight [ 32 P]-labeled RNAs ( Fig. 3e ). Thus, a single acetylation-mimic mutation at Lys-145 within RRM1 is sufficient to significantly impair TDP-43 binding to its cellular mRNA targets. Arsenite-induced oxidative stress induces TDP-43 acetylation Given that TDP-43 has high-affinity RNA binding under normal conditions [46] , [47] , we hypothesized that accessibility to target lysines would occur more readily following detachment of TDP-43 from RNAs. Therefore, we employed an oxidative stress paradigm in which sodium arsenite treatment was previously shown to impair TDP-43 binding to RNAs, leading to loss of function and insoluble TDP-43 accumulation [11] . Supporting stress-induced loss of TDP-43 function, acute arsenite exposure promoted rapid accumulation of TDP-43-ΔNLS into phosphorylated cytoplasmic inclusions, while WT TDP-43 formed insoluble nuclear foci that were not phosphorylated ( Fig. 4a ). Quantification of these results indicated that cytoplasmic TDP-43 showed a slightly increased propensity to undergo stress-induced re-localization and aggregation compared with WT nuclear TDP-43 ( Fig. 4b ). Therefore, either oxidative stress or TDP-43 acetylation is capable of promoting TDP-43 aggregation and loss of function ( Figs 2b and 4b ), suggesting a common signalling pathway in which oxidative stress could mediate TDP-43 acetylation and subsequent aggregation. 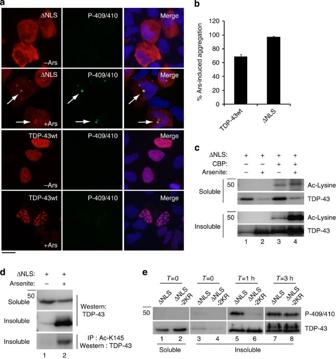Figure 4: Oxidative stress promotes TDP-43 acetylation and pathological TDP-43 aggregation. (a) Double-labelling immunofluorescence microscopy of WT TDP-43 or cytoplasmic TDP-43 was performed using anti-myc and anti-phospho-TDP-43 (P-409/410) antibodies, which illustrate TDP-43 phosphorylation and aggregation on acute exposure to 0.2 mM arsenite for 1 h. Scale bar, 25 μm. (b) Quantification of nuclear or cytoplasmic TDP-43 stippling and aggregation phenotypes for all lysine mutants was performed fromN=3 independent experiments as detailed in the Methods section. Error bars represent s.e.m. (c) Immunoblotting of soluble and insoluble fractions using anti-myc and anti-acetyl-lysine antibodies illustrates the accumulation of acetylated TDP-43 on co-transfection of CBP and exposure to 0.2 mM arsenite for 1 h. (d) Immunoprecipitation reaction using Ac-K145 followed by immunoblotting with a monoclonal anti-TDP-43 antibody allowed increased sensitivity for detection of acetylated TDP-43 in the absence of CBP (see alsoSupplementary Fig. 11). (e) Immunoblotting analysis of TDP-43-ΔNLS and the double lysine mutant, TDP-43-ΔNLS-2KR, was evaluated in an arsenite-induced aggregation time-course, which showed delayed accumulation of phosphorylated TDP-43-ΔNLS-2KR aggregates compared with TDP-43-ΔNLS. Figure 4: Oxidative stress promotes TDP-43 acetylation and pathological TDP-43 aggregation. ( a ) Double-labelling immunofluorescence microscopy of WT TDP-43 or cytoplasmic TDP-43 was performed using anti-myc and anti-phospho-TDP-43 (P-409/410) antibodies, which illustrate TDP-43 phosphorylation and aggregation on acute exposure to 0.2 mM arsenite for 1 h. Scale bar, 25 μm. ( b ) Quantification of nuclear or cytoplasmic TDP-43 stippling and aggregation phenotypes for all lysine mutants was performed from N =3 independent experiments as detailed in the Methods section. Error bars represent s.e.m. ( c ) Immunoblotting of soluble and insoluble fractions using anti-myc and anti-acetyl-lysine antibodies illustrates the accumulation of acetylated TDP-43 on co-transfection of CBP and exposure to 0.2 mM arsenite for 1 h. ( d ) Immunoprecipitation reaction using Ac-K145 followed by immunoblotting with a monoclonal anti-TDP-43 antibody allowed increased sensitivity for detection of acetylated TDP-43 in the absence of CBP (see also Supplementary Fig. 11 ). ( e ) Immunoblotting analysis of TDP-43-ΔNLS and the double lysine mutant, TDP-43-ΔNLS-2KR, was evaluated in an arsenite-induced aggregation time-course, which showed delayed accumulation of phosphorylated TDP-43-ΔNLS-2KR aggregates compared with TDP-43-ΔNLS. Full size image To investigate this possibility, biochemical analysis showed that insoluble TDP-43-ΔNLS aggregates became increasingly acetylated on co-transfection of CBP and exposure to acute arsenite stress ( Fig. 4c , lanes 3–4 and Supplementary Fig. 9 ). To assess whether stress-induced TDP-43 acetylation could occur in the absence of ectopically expressed CBP acetyltransferase, we generated a site-specific acetylated TDP-43 antibody against Lys-145 to increase the specificity and detection sensitivity for acetylated TDP-43 (referred to as Ac-K145, see Supplementary Fig. 10 for antibody characterization). Ac-K145 did not reliably detect acetylated TDP-43 by direct immunoblot analysis of insoluble lysates; however, we found that Ac-K145 immunoprecipitated acetylated TDP-43 from insoluble fractions of arsenite-treated cells, and was then detected by immunoblotting with total TDP-43 antibodies ( Fig. 4d , lane 2 and Supplementary Fig. 11 ). To assess the aggregation propensity of a non-acetylated mutant at Lys-145 and Lys-192 (TDP-43-ΔNLS-2KR) in response to arsenite stress, a time-course analysis of TDP-43 aggregation was performed, which showed a delay in the progressive accumulation of phosphorylated TDP-43 species (P-409/410) ~1 h after arsenite exposure ( Fig. 4e , lanes 5–6, and Supplementary Fig. 11 ), suggesting acetylation at these specific lysines could contribute to stress-induced maturation of TDP-43 aggregates. Thus, potent oxidative stressors can act as environmental signals to induce acetylation, aggregation and loss of critical TDP-43 functions. HDAC6 interacts with and deacetylates TDP-43 As our data suggest that acetylation promotes TDP-43 aggregation, we sought to identify a TDP-43 deacetylase capable of regulating this process. One potential candidate is the cytoplasmic deacetylase HDAC6, previously implicated in the clearance of misfolded protein aggregates in several neurodegenerative diseases [48] , [49] , [50] , [51] , [52] , [53] , [54] , [55] , [56] , [57] . A more recent study demonstrated a direct physical interaction between HDAC6 and TDP-43 in vivo [58] . Therefore, we evaluated whether HDAC6 regulates TDP-43 acetylation and aggregation. Co-expression of WT HDAC6, but not a catalytically inactive H803A mutant, together with CBP was sufficient to deacetylate cytoplasmic TDP-43 under normal cellular conditions ( Fig. 5a , lanes 2–4 and Supplementary Fig. 12 ). Moreover, co-immunoprecipitation experiments revealed an interaction between cytoplasmic TDP-43 and HDAC6 that was enhanced on exposure to arsenite stress, but not a less potent oxidative stress induced by hydrogen peroxide ( Fig. 5b and Supplementary Fig. 13 ). The arsenite-induced TDP-43–HDAC6 interaction was rather unexpected, as HDAC6 recruitment during arsenite exposure was not sufficient to promote TDP-43 deacetylation (see Fig. 4c,d ), suggesting an inability of cytoplasmic TDP-43 aggregates to become efficiently deacetylated by HDAC6. Confirming HDAC6 recruitment to TDP-43 aggregates, both acetylation-mimic (TDP-43-ΔNLS-K145Q) and arsenite-induced acetylated TDP-43 aggregates physically interacted with HDAC6 by co-immunoprecipitation assays ( Fig. 5c , lanes 2–4 and Supplementary Fig. 13 ) and also co-localized with ectopically expressed or endogenous HDAC6 protein ( Fig. 5d ). Notably, cytoplasmic TDP-43 aggregates also recruited and activated the CHIP/Hsp70 complex ( Fig. 5e and Supplementary Figs 14 and 15 ), previously implicated together with HDAC6 in the targeted clearance of the microtubule-associated tau protein [48] , [59] , [60] . 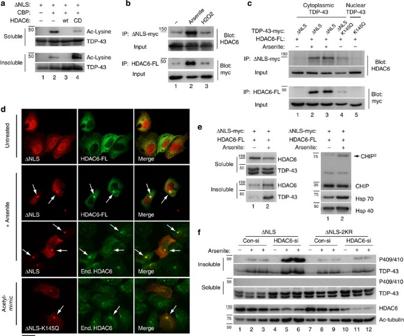Figure 5: The deacetylase HDAC6 binds and deacetylates TDP-43 in a stress-regulated manner. (a) Cells were co-transfected with TDP-43-ΔNLS, CBP, and either wild-type HDAC6 or the catalytically dead HDAC6-H611A mutant and TDP-43 acetylation was determined by immunoblotting with acetyl-lysine antibodies similar toFig. 1c. (b) Cells transfected with myc-tagged TDP-43-ΔNLS and FLAG-tagged HDAC6 were analysed by co-immunoprecipitation reactions under basal or stimulated conditions in the presence of 0.1 mM arsenite or 1 mM peroxide stress for 2 h. Input, representing 5% of total lysate volume, was analysed by immunoblotting using the indicated antibodies. (c) Co-immunoprecipitation analysis using either TDP-43-ΔNLS or acetylation mimic mutants (TDP-43-K145Q or TDP-43-ΔNLS-K145Q) and wild-type HDAC6 was performed in the absence or presence of arsenite, and immunoprecipitated proteins were analysed by western blotting with the indicated antibodies similar tobabove. (d) Immunofluorescence microscopy was performed on cells expressing myc-tagged TDP-43-ΔNLS, acetylation mimic TDP-43-ΔNLS-K145Q and HDAC6-FLAG where indicated, using anti-FLAG or endogenous HDAC6 antibodies. TDP-43 acetylation-mimic mutations or acute treatment with arsenite led to the formation of cytoplasmic aggregates that co-localized with HDAC6. Scale bar, 25 μm. (e) Protein levels of the HDAC6/CHIP/Hsp70 complex were determined by western analysis of soluble and insoluble fractions using HDAC6, CHIP, Hsp70 and Hsp40 specific antibodies. Note, CHIP dimers (arrowhead) suggest activation of CHIP E3 ligase function, as previously reported68. (f) Depletion of HDAC6 was performed using a specific HDAC6 siRNA followed by arsenite treatment, and solubility of TDP-43-ΔNLS and TDP-43-ΔNLS-2KR proteins was analysed by immunoblotting with total and phosphorylated TDP-43 antibodies. HDAC6 siRNA knockdown efficiency was validated by assessing total levels of HDAC6 and its major substrate acetylated tubulin. Figure 5: The deacetylase HDAC6 binds and deacetylates TDP-43 in a stress-regulated manner. ( a ) Cells were co-transfected with TDP-43-ΔNLS, CBP, and either wild-type HDAC6 or the catalytically dead HDAC6-H611A mutant and TDP-43 acetylation was determined by immunoblotting with acetyl-lysine antibodies similar to Fig. 1c . ( b ) Cells transfected with myc-tagged TDP-43-ΔNLS and FLAG-tagged HDAC6 were analysed by co-immunoprecipitation reactions under basal or stimulated conditions in the presence of 0.1 mM arsenite or 1 mM peroxide stress for 2 h. Input, representing 5% of total lysate volume, was analysed by immunoblotting using the indicated antibodies. ( c ) Co-immunoprecipitation analysis using either TDP-43-ΔNLS or acetylation mimic mutants (TDP-43-K145Q or TDP-43-ΔNLS-K145Q) and wild-type HDAC6 was performed in the absence or presence of arsenite, and immunoprecipitated proteins were analysed by western blotting with the indicated antibodies similar to b above. ( d ) Immunofluorescence microscopy was performed on cells expressing myc-tagged TDP-43-ΔNLS, acetylation mimic TDP-43-ΔNLS-K145Q and HDAC6-FLAG where indicated, using anti-FLAG or endogenous HDAC6 antibodies. TDP-43 acetylation-mimic mutations or acute treatment with arsenite led to the formation of cytoplasmic aggregates that co-localized with HDAC6. Scale bar, 25 μm. ( e ) Protein levels of the HDAC6/CHIP/Hsp70 complex were determined by western analysis of soluble and insoluble fractions using HDAC6, CHIP, Hsp70 and Hsp40 specific antibodies. Note, CHIP dimers (arrowhead) suggest activation of CHIP E3 ligase function, as previously reported [68] . ( f ) Depletion of HDAC6 was performed using a specific HDAC6 siRNA followed by arsenite treatment, and solubility of TDP-43-ΔNLS and TDP-43-ΔNLS-2KR proteins was analysed by immunoblotting with total and phosphorylated TDP-43 antibodies. HDAC6 siRNA knockdown efficiency was validated by assessing total levels of HDAC6 and its major substrate acetylated tubulin. Full size image These results suggested that HDAC6-mediated deacetylation of TDP-43 may represent a homeostatic response to alleviate the burden of TDP-43 aggregates. To address this possibility, we analysed arsenite-induced aggregation of cytoplasmic TDP-43 in the absence of HDAC6 using siRNA-mediated gene silencing. HDAC6 siRNA led to an increase in arsenite-stimulated TDP-43-ΔNLS aggregation, which was reflected by an increase in both total TDP-43 as well as phosphorylated TDP-43 recovered in insoluble fractions ( Fig. 5f , compare lanes 2–3 with lanes 5–6 and Supplementary Fig. 16 ). Importantly, the effect of HDAC6 on insoluble TDP-43 accumulation was dependent on Lys-145 and Lys-192 acetylation sites, as loss of HDAC6 did not promote comparable aggregation of a TDP-43-ΔNLS-2KR mutant lacking those critical lysine residues ( Fig. 5f , compare lanes 8–9 with lanes 11–12). Taken together, these data suggest that, although HDAC6 can deacetylate TDP-43 under basal conditions, exposure to oxidative stress promotes the formation of TDP-43 aggregates that are not effectively deacetylated and thereby accumulate as mature aggregated TDP-43 species. Acetylated TDP-43 inclusions are linked to ALS To investigate TDP-43 acetylation in human TDP-43 proteinopathies, immunohistochemistry (IHC) was performed on human brain and spinal cord tissues from subjects with frontotemporal dementia with TDP-43 pathology (FTLD-TDP) and ALS (see Table 1 for case demographics), both of which are characterized by robust TDP-43 pathology. As expected, the FTLD-TDP brain contained strongly P-409/410-immunoreactive TDP-43 inclusions ( Fig. 6a ), which were not readily detectable with an Ac-K145 antibody ( Fig. 6b and Table 1 ), indicating a lack of TDP-43 acetylation at Lys-145 in FTLD-TDP. However, given that pathological TDP-43 species in FTLD-TDP were shown to consist predominantly of C-terminal truncated fragments beginning with residue Arg-208 (ref. 40 ), we speculated that TDP-43 fragmentation in the FTLD-TDP brain would preclude the detection of TDP-43 acetylation on Lys-145 as this residue is not present in the cleaved pathological TDP-43 fragment. Table 1 Demographics of human FTLD-TDP and ALS cases used in this study. 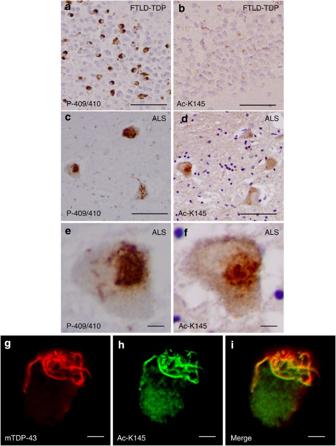Figure 6: TDP-43 acetylation is a pathological feature of ALS but not FTLD-TDP. (a–f) Immunohistochemistry (IHC) was performed on cortical brain and spinal cord sections from frontotemporal dementia (FTLD-TDP) and ALS cases that harbour abundant TDP-43 pathology. Shown are representative images of TDP-43 inclusions detected with phosphorylated (P-409/410) and acetylated (Ac-K145) TDP-43 antibodies. FTLD-TDP inclusions showed characteristic phosphorylated TDP-43 immunoreactivity with P-409/410 (a), which was not detected with Ac-K145 (b). Serial ALS spinal cord sections analysed by IHC identified TDP-43 inclusions that were immunoreactive with both P409/410 (c,e) and Ac-K145 antibodies (d,f), indicating acetylation of TDP-43 in ALS spinal cord lesions. SeeTable 1for a summary of P-409/410 and Ac-K145 immunoreactivity and details of ALS cases used in this study. (g–i) Double-labelling immunofluorescence was performed on ALS spinal cord sections using monoclonal anti-TDP-43 (panelg, red) and Ac-K145 (panelh, green) antibodies. The merged image (paneli) highlights the co-localization observed between total TDP-43 and acetylated TDP-43. Scale bar, 50 μm (panelsa–d) and 10 μm (panelse,fandg–i). Full size table Figure 6: TDP-43 acetylation is a pathological feature of ALS but not FTLD-TDP. ( a – f ) Immunohistochemistry (IHC) was performed on cortical brain and spinal cord sections from frontotemporal dementia (FTLD-TDP) and ALS cases that harbour abundant TDP-43 pathology. Shown are representative images of TDP-43 inclusions detected with phosphorylated (P-409/410) and acetylated (Ac-K145) TDP-43 antibodies. FTLD-TDP inclusions showed characteristic phosphorylated TDP-43 immunoreactivity with P-409/410 ( a ), which was not detected with Ac-K145 ( b ). Serial ALS spinal cord sections analysed by IHC identified TDP-43 inclusions that were immunoreactive with both P409/410 ( c , e ) and Ac-K145 antibodies ( d , f ), indicating acetylation of TDP-43 in ALS spinal cord lesions. See Table 1 for a summary of P-409/410 and Ac-K145 immunoreactivity and details of ALS cases used in this study. ( g–i ) Double-labelling immunofluorescence was performed on ALS spinal cord sections using monoclonal anti-TDP-43 (panel g , red) and Ac-K145 (panel h , green) antibodies. The merged image (panel i ) highlights the co-localization observed between total TDP-43 and acetylated TDP-43. Scale bar, 50 μm (panels a – d ) and 10 μm (panels e , f and g – i ). Full size image To further examine Lys-145 acetylation in TDP-43 proteinopathies, we analysed the ALS spinal cord, which, in contrast to FTLD-TDP, harbours significant TDP-43 pathology that consists predominantly of full-length TDP-43, as both N- and C-terminal TDP-43 antibodies are capable of detecting TDP-43 inclusions in ALS motor neurons [28] . Therefore, pathological TDP-43 species in the ALS spinal cord should contain the targeted Lys-145 acetylation site. Using serial spinal cord sections from ALS patients, we detected robust P-409/410 immunoreactive inclusions ( Fig. 6 , panels c and e), and most of the phosphorylated TDP-43 lesions also showed significant skein-like Ac-K145 immunoreactivity ( Fig. 6 , panels d and f, and Table 1 ). To confirm that Ac-K145 detected TDP-43-positive inclusions in the ALS spinal cord, double-labelling immunofluorescence revealed substantial co-localization of acetylated TDP-43 (Ac-K145) with total TDP-43, as detected with a human-specific monoclonal TDP-43 antibody ( Fig. 6 , panels g–i). These results reveal that acetylated TDP-43 is a pathological feature associated with full-length, phosphorylated TDP-43 lesions in the ALS spinal cord but not the FTLD-TDP brain and support acetylation-induced loss of TDP-43 function and aggregation as a potential pathogenic mechanism in ALS and possibly other TDP-43 proteinopathies. In this study, we have identified TDP-43 acetylation as a novel post-translational modification regulating TDP-43 functional and biochemical properties. Although WT nuclear TDP-43 is also subject to acetylation, we found increased cytoplasmic TDP-43 acetylation, possibly due to enhanced lysine accessibility or conformational differences between nuclear and cytoplasmic TDP-43. Given that TDP-43 primarily forms cytoplasmic inclusions in the diseased brain and spinal cord, we speculate that increased acetylation in the cytoplasm could be responsible, in part, for inclusion formation in TDP-43 proteinopathies. Indeed, using an acetylation-specific antibody (Ac-K145), we detected acetylated TDP-43 pathology in the ALS spinal cord, suggesting TDP-43 acetylation is linked to ALS pathogenesis ( Fig. 6 ). Supporting a pathological role, acetylation at Lys-145 was sufficient to increase TDP-43 pathogenicity in cells, as determined by both nuclear and cytoplasmic TDP-43 aggregation, increased C-terminal TDP-43 phosphorylation and loss of normal nuclear TDP-43 function. Thus, we propose that aberrant TDP-43 acetylation can act in a pathogenic manner to trigger aggregation and loss of TDP-43 function (see Fig. 7 model). Future studies are required to determine whether TDP-43 acetylation is limited to ALS or whether this modification occurs in a range of other TDP-43 proteinopathies, potentially expanding the clinical and therapeutic relevance of this finding. 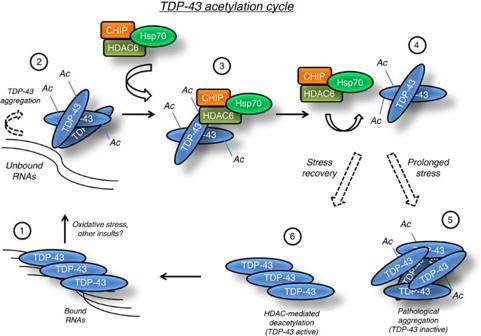Figure 7: Model for reversible regulation of TDP-43 via lysine acetylation. TDP-43 binds with high affinity to nucleic acids under normal cellular conditions (step 1). Oxidative stress and potentially other environmental or genetic insults promote cysteine disulfide crosslinking11and lysine acetylation (this study), which abrogate binding to TDP-43 target RNAs leading to the accumulation of unbound TDP-43 in the nucleus and cytoplasm (step 2). Free unbound TDP-43 is susceptible to lysine acetylation within the RNA-binding domain on Lys-145 and Lys-192, which prevents TDP-43 association with target RNAs and promotes TDP-43 aggregation most readily in the cytoplasmic compartment (Fig. 2). Acetylated TDP-43 aggregates are readily engaged by an HDAC6/CHIP/Hsp70 complex (step 3) that is capable of deacetylating TDP-43 under normal conditions (step 4), but not during sustained exposure to potent oxidative stimuli (step 5), the latter of which favours the formation of pathological full-length and acetylated TDP-43 lesions that are detectable in the ALS spinal cord (Fig. 6). TDP-43 deacetylation conversely would result in engagement of TDP-43 mRNA targets, stabilization of TDP-43 conformation, and re-establishment of normal TDP-43 function as an active RNA regulatory protein (step 6, return to step 1). Figure 7: Model for reversible regulation of TDP-43 via lysine acetylation. TDP-43 binds with high affinity to nucleic acids under normal cellular conditions (step 1). Oxidative stress and potentially other environmental or genetic insults promote cysteine disulfide crosslinking [11] and lysine acetylation (this study), which abrogate binding to TDP-43 target RNAs leading to the accumulation of unbound TDP-43 in the nucleus and cytoplasm (step 2). Free unbound TDP-43 is susceptible to lysine acetylation within the RNA-binding domain on Lys-145 and Lys-192, which prevents TDP-43 association with target RNAs and promotes TDP-43 aggregation most readily in the cytoplasmic compartment ( Fig. 2 ). Acetylated TDP-43 aggregates are readily engaged by an HDAC6/CHIP/Hsp70 complex (step 3) that is capable of deacetylating TDP-43 under normal conditions (step 4), but not during sustained exposure to potent oxidative stimuli (step 5), the latter of which favours the formation of pathological full-length and acetylated TDP-43 lesions that are detectable in the ALS spinal cord ( Fig. 6 ). TDP-43 deacetylation conversely would result in engagement of TDP-43 mRNA targets, stabilization of TDP-43 conformation, and re-establishment of normal TDP-43 function as an active RNA regulatory protein (step 6, return to step 1). Full size image To elucidate possible physiological consequences of acetylation as it relates to normal TDP-43 biology, we investigated nucleo-cytoplasmic shuttling, TDP-43 protein stability and TDP-43 association with target RNAs. Immunofluorescence experiments demonstrated that acetylation did not significantly alter TDP-43 nucleo-cytoplasmic shuttling, as acetylated TDP-43 was retained in its respective subcellular compartments, albeit with altered morphology as discrete nuclear foci and cytoplasmic aggregates ( Fig. 2a ). Acetylation also did not significantly alter steady–state TDP-43 protein levels in our cell-based system, suggesting a minimal effect of acetylation on TDP-43 half-life. This is in contrast to acetylation-induced protein degradation observed with the Huntingtin (Htt) protein [61] . Finally, we evaluated whether acetylation altered association with target mRNAs, as our mass spectrometry data identified acetylation on Lys-145 and Lys-192 within the RRM domains of TDP-43 ( Fig. 1g,h ). Indeed, our results suggest that a single acetylation event is sufficient to impair RNA binding and splicing function ( Fig. 3 ), implicating Lys-145 as a critical determinant of TDP-43 function. These data are consistent with a recent study showing that non-specific chemical acetylation of Lys-145 in vitro using acetic anhydride occurred most efficiently in the absence of RNA, suggesting that RNA binding protects Lys-145 from acetylation [46] . Taken together, we conclude that TDP-43 acetylation within the RRMs is sufficient to impair normal RNA binding ( Fig. 7 , step 2), thereby providing a rapid and efficient regulatory switch to modulate TDP-43 association with downstream target RNAs. Our previous study demonstrated that TDP-43 is subject to redox regulation, in which oxidative stress promotes TDP-43 cysteine oxidation and disulfide crosslinking, which prevents RNA binding and splicing function [11] . As our current study showed that oxidative stress also promotes TDP-43 acetylation, it is conceivable that cysteine oxidation and lysine acetylation represent two critical modifications that coordinately regulate TDP-43 function under stress conditions, although the temporal sequence of these modifications still remains unclear. However, as redox sensing is generally a rapidly transduced signal, cysteine oxidation and partial loss of RNA binding could initially provide increased accessibility for subsequent lysine acetylation within the RRMs and would support a ‘multiple hit’ model previously suggested for TDP-43 pathogenesis [2] , [11] . Once disengaged from its targets, TDP-43 likely assumes an inherently unstable conformation that is highly aggregation-prone [11] , [62] , [63] , and therefore we hypothesized that acetylation alone would be sufficient to trigger loss of RNA binding and increased aggregation propensity. Indeed, acetylation conferred by the acetyltransferase CBP or acetylation-mimic mutations was sufficient to induce loss of RNA binding and the accumulation of insoluble and phosphorylated TDP-43 ( Fig. 2 ). Future studies are required to elucidate the cross-talk among multiple TDP-43 modifications (cysteine oxidation, acetylation, phosphorylation, ubiquitination and C-terminal cleavage) and their individual contributions to TDP-43 function and aggregation. Regardless of the detailed sequence of events, our results reveal that a complex post-translational signalling cascade is likely involved in TDP-43 pathogenesis. Cellular defense mechanisms exist to re-fold or clear potentially toxic aggregated species, which, if defective, may contribute to the pathogenesis of ALS [64] , [65] . We speculate that elevated deacetylase activity may act in this regard to reduce TDP-43 aggregation, and thereby maintain active TDP-43 that is essential for cell survival. As a recent study identified a physical interaction between TDP-43, HDAC6, and Parkin in vivo that may regulate TDP-43 cytoplasmic accumulation [58] , we focused on HDAC6 as one potential regulator of TDP-43 acetylation and aggregation. Interestingly, while HDAC6 was sufficient to deacetylate soluble cytoplasmic TDP-43, we observed that cytoplasmic TDP-43 aggregates were unable to be efficiently deacetylated, possibly due to limited accessibility to lysines that are buried within the RRM-containing aggregates. Thus, an inability of HDAC6 and related quality control machinery to effectively deacetylate TDP-43 could lead to increased TDP-43 aggregation and contribute, in part, to disease pathogenesis similar to that proposed for abnormal tau acetylation in Alzheimer’s disease [31] , [33] , [34] , [35] . In support of this pathogenic mechanism, loss of HDAC6 exacerbated TDP-43 aggregation and led to an increase in insoluble and phosphorylated TDP-43 ( Fig. 5f ). Conversely, we predict that future approaches to reduce levels of acetylated TDP-43, for example by pharmacologically targeting putative TDP-43 acetyltransferase(s), might allow increased RNA binding and enhancement of critical TDP-43 nuclear functions ( Fig. 7 , step 6). Overall, the identification of a reversible TDP-43 acetylation switch provides a novel framework to further understand both physiological and pathological TDP-43 functions, which could lead to targeted therapies against ALS and related TDP-43 proteinopathies. Plasmids and cell culture Human TDP-43 was cloned into pCDNA5/TO vector (Invitrogen) and site-directed mutagenesis (Quikchange kit; Stratagene) was used to create K→Q or K→R mutations at residues K145 and K192 as indicated. Creb-binding protein (CBP) plasmids as well as WT-HDAC6 and HDAC6-H803A enzyme-inactive mutant expression plasmids were kindly provided by Dr Tso-Pang Yao (Duke University). Plasmids were transfected into QBI-293 cells (MP Biomedicals) using Fugene 6 (Roche) per manufacturer’s instructions. HDAC6 siRNA (Invitrogen) sequence was as follows: 5′- AAAGUUGGAACUCUCACGGUGCAGC -3′ and was transfected using RNAi Max reagent (Invitrogen) following the manufacturer’s protocols. For oxidative stress treatments, confluent QBI-293 cells grown in six-well or 10cm dishes were exposed to 50 μM sodium arsenite or 1 mM hydrogen peroxide for 1–12 h, as indicated in text. Cells were harvested and analysed by western blotting using the indicated antibodies, as detailed below. Mouse Neuro2A neuroblastoma cells (ATCC) were transfected using Fugene 6 with ▵ NLS, ▵ NLS-K145Q and ▵ NLS-2KQ plasmids and differentiated by 24 h withdrawal of fetal bovine serum (FBS), which promotes extension of neuritic processes, followed by subsequent western blotting and immunofluorescence studies. Splicing assay TDP-43 functional activity was assessed using a tandem transfection CFTR splicing assay. Either control (pcDNA‐5TO vector), TDP-43 shRNA construct (Origene), wild-type (WT) TDP-43, TDP-K145Q or TDP-4FL mutants were transiently transfected into QBI‐293 cells using Lipofectamine 2000 reagent (Invitrogen) following the standard manufacturer’s protocols. After 48 h, a hybrid minigene construct TG(13)T(5) (a generous gift from Dr F Baralle, International Centre for Genetic Engineering and Biotechnology, Trieste, Italy), which monitors CFTR exon 9 splicing, was transiently transfected into the same cells. Twenty-four hours after minigene transfection, cells were harvested, and CFTR exon 9 inclusion versus exclusion in the presence of the indicated TDP-43 plasmids was then evaluated by RT–PCR from isolated total RNA prepared from cells 72 h after transfection of TDP-43 constructs and 24 h after transfection of the TG(13)T(5) CFTR minigene reporter construct. The RT-PCR primers were as follows: Bra2, 5′- TAGGATCCGGTCACCAGGAAGTTGGTTAAATCA -3′; a2–3, 5′- CAACTTCAAGCTCCTAAGCCACTGC -3′. PCR conditions were as follows: 95 °C for 10 min (hot start), followed by 30 cycles of denaturing at 95 °C for 30 s, annealing at 57 °C for 30 s and elongation at 72 °C for 60 s. PCR products were visualized on a 1.5% agarose gel and Exon 9 splice products were quantified using the Agilent 2100 Bioanalyzer on a DNA 1000 chip and values were calculated as log ratios of spliced/unspliced products. Crosslinking immunoprecipitation assay Cell-based crosslinking immunoprecipitation (CLIP) assay was performed similar to that described [66] , [67] with minor variations. Transfected QBI-293 cells grown in a 10-cm dish were UV irradiated twice consecutively in 5 ml cold PBS at 400 mJ cm −2 . Cells were pelleted and stored at −80 until use. Cell pellets were lysed in NP-40 lysis buffer (50 mM Tris-HCL, pH 7.5; 150 mM NaCl, 0.5% NP-40, 50 mM NaF containing RNAsin (Promega) and incubated 10 min on ice followed by addition of RQ1 DNase (Promega, M6101; 30 U) to each tube and incubated at 37 °C for 5 min. RNase A (USB #70194Y) was added at 1:5,000 dilution and incubated at 37 °C for 5 min, followed by ultra-centrifugation with polycarbonate tubes at 30,000 r.p.m. for 20 min at 4 °C. The supernatant containing TDP-43 bound RNAs was mixed with protein A/G beads (Santa Cruz) and 5 μg anti-myc 9E10 antibody (Santa Cruz) and rotated 3–4 h 4 °C. Beads were washed as follows: two times with ice-cold NP-40 lysis buffer, two times with buffer B [5 × PBS (no Mg 2+ , no Ca 2+ ), 0.5% NP-40] and two times with buffer C (50 mM Tris–Cl, pH 7.4, 10 mM MgCl 2 , 0.5% NP-40). TDP-43 bound A/G beads were then treated with Calf-Intestinal Alkaline Phosphatase (NEB) in the presence of RNAs according to the manufacturer’s protocol. Samples were washed once with Buffer C (see above), once with Buffer D (50 mM Tris-HCL, pH 7.5; 20 mM EGTA; 0.5% NP-40) and then twice with Buffer C. RNAs were end-labelled using [ 32 P]- γ- ATP (Perkin Elmer, BLU002A) and T4 PNK enzyme (NEB, T4 polynucleotide kinase, M0201L) followed by bead washes: once with NP-40 lysis buffer, twice with Buffer B and five times with buffer C. Samples were loaded onto 10% Bis-Tris gels (Bio-Rad) using an MOPS running buffer system, transferred onto nitrocellulose membranes and signals were quantified as pixel intensities using a TYPHOON phosphorimager system and normalized to WT TDP-43 bound RNAs. Recombinant TDP-43 methods TDP-43 recombinant proteins (WT, K145/192Q, K145/192R) were purified from BL-21 cells using the pCOLD vector expression system (Takara Bio). After protein induction, all TDP-43 proteins were present predominantly in insoluble fractions of bacterial lysates. To generate soluble-purified TDP-43 protein, bacterial pellets were washed extensively 5 × in RIPA buffer to remove soluble proteins, and insoluble pellets containing TDP-43 proteins were subsequently extracted repeatedly in 0.1% SDS, 0.1 M MOPS pH 7.5 and TDP-43 solubility was monitored until total protein was solubilized. Re-solubilized TDP-43 proteins were estimated to be ~95% pure based on visualization by Coomassie staining. Protein stocks were maintained at high concentration (10 mg ml −1 ) in 0.1% SDS, 0.1 M MOPS pH 7.5 to prevent loss of TDP-43 solubility. We note that TDP-2KQ mutant protein required repetitive extractions in 0.1% SDS, 0.1 M MOPS pH 7.5 to re-solubilize the protein, indicating reduced solubility due to impaired binding to nucleic acids. Peptide/antibody generation Polyclonal anti-acetyl TDP-43 (K145) antibodies were generated using the acetylated TDP-43 peptide GHSKGFG-C containing K145 acetylation which was used to immunize rabbits (Pocono Rabbit Farm and Laboratory, Canadensis, PA). Double affinity purification was performed using native and acetylated peptides sequentially using Sulfolink columns (Pierce Biotechnology). Site specificity of Ac-K145 was confirmed in vitro by western blot analysis of purified WT and lysine mutant proteins (see above) and by peptide ELISA assays using acetylated and unmodified peptides ( Supplementary Fig. 10 ). Biochemical methods and co-immunoprecipitation analysis Fractionation of all cell lysates was performed by sequential extraction using buffers of increasing strength. Cells from six-well culture dishes were scraped into 300 ml RIPA buffer (50 mM Tris pH 8.0, 150 mM NaCl, 1%NP-40, 5 mM EDTA, 0.5% sodium deoxycholate, 0.1%SDS) containing 1 mM phenylmethylsulfonyl fluoride, a mixture of protease inhibitors (1 mg ml −1 pepstatin, leuptin, N -p-tosyl-L-phenylalanine chloromethyl ketone, Nα-Tosyl-L-lysine chloromethyl ketone hydrochloride, trypsin inhibitor; Sigma) and a mixture of phosphatase inhibitors (2 mm imidazole, 1 mm NaF, 1 mm sodium orthovanadate; Sigma). Samples were sonicated and centrifuged at 100,000 g for 30 min at 4 °C, and then re-extracted in RIPA buffer to ensure complete removal of soluble proteins. Resultant insoluble pellets were extracted in urea buffer (7 M urea, 2 M Thiourea, 4%CHAPS, 30 mM Tris, pH 8.5), sonicated and centrifuged at 100,000 × g for 30 min at room temperature. Soluble and insoluble fractions were analysed by western blotting using the indicated antibodies. Antibodies for western analysis were as follows: rabbit polyclonal anti-TDP-43 (Proteintech) 1:1,000, mouse monoclonal antibody anti-TDP-43 (Proteintech) 1:1,000, rabbit polyclonal anti-TDP-43 C-terminal 1038 1:10,000, rabbit polyclonal anti-TDP-43 N-terminal 1065 1:10,000, anti-GAPDH (6C5 mouse mAb; Advanced ImmunoChemical) 1:3,000, anti-acetylated tubulin (Sigma) 1:1,000, anti-α-tubulin (Sigma) 1:1,000, anti-HDAC6 (H-300; Santa Cruz) 1:1,000, anti-acetyl-lysine (1:1,000, Cell Signalling), polyclonal anti-CHIP (1:1,000, Sigma). For insoluble Ac-K145 immunoprecipitation reactions, urea solubilized fractions were diluted tenfold in Triton buffer (1% Triton-X-100, 40 mM Tris pH 8.0) before immunopreciptation reactions using 10 μg of Ac-K145 antibody conjugated to protein A/G beads, followed by extensive washes and western blotting using a monoclonal TDP-43 antibody (Proteintech). For co-immunoprecipitation studies, QBI-293 cells were lysed in NP-40 lysis buffer referred to as NETN buffer (50 mM Tris-Cl, pH 7.4, 150 mM NaCl, 1 mM EDTA, 1% NP-40, 1 mM sodium orthovanadate, 1 mM sodium fluoride, 1 mM PMSF, 0.2 mM leupeptin, protease inhibitor cocktail). Soluble supernatants (1 mg total protein) were cleared by centrifugation, incubated overnight with protein A/G beads (Santa Cruz) complexed to the indicated antibodies described in the figure legends, and subsequently analysed by SDS–PAGE and immunoblotting. Immunoprecipitation and mass spectrometry analysis For cell-based mass spectrometry (MS) analysis, 10-cm dishes of QBI-293 cells were transiently transfected with TDP-43-ΔNLS and CBP plasmids. Total lysates were prepared and TDP-43 was immunoprecipitated from these fractions using anti-TDP-43 (clone 171) complexed to protein A/G beads (Sigma). Immunoprecipitated samples were analysed by SDS–PAGE electrophoresis in the presence of reducing agents and analysed by Coomassie staining and gel excision followed by nanoLC/nanospray/MS/MS. The analysis was performed using the University of Pennsylvania proteomics core facility and data were acquired with Xcalibur 2.0 (ThermoFisher) and analysed with PEAKS 6.0 (Bioinformatics Solutions) and Scaffold 3 (Proteome Software) software packages. Cutoffs: peptide P -value <95%; protein P -value <99.0%. Immunocytochemistry and quantification Cultured cells were fixed in 4% paraformaldehyde (PFA) for 10 min, rinsed three times in PBS and permeabilized with 0.2% Triton X-100 (Sigma) in PBS for 10 min. Cells were then blocked in 5% milk for 1 h and subsequently incubated with primary antibodies of interest overnight at 4 °C following standard immunofluorescence techniques. Cell-based nuclear stippling and cytoplasmic aggregation of lysine mutants was performed by immunofluorescence microscopy (× 40 magnification) using an Olympus BX 51 microscope. Stippling and aggregation phenotypes were quantified as a percent of transfected cells using >10 fields, and sampling error was calculated using the s.e.m. Statistical analysis was determined using a two-tailed unpaired t -test with unequal variance (significance set at P -values <0.05). All quantitative fluorescence was independently validated with a minimum of N =3 biological replicates. Primary antibodies used for immunofluorescence were as follows: polyclonal anti-TDP-43 (Proteintech, 1:500), polyclonal anti-myc (1:4,000, Sigma), monoclonal anti-myc 9E10 (Sigma, 1:1,000), monoclonal anti-Hsp70 (Stressgen, 1:500). Immunohistochemistry and double labelling For human studies, fixed, paraffin-embedded tissue blocks were obtained from the Center for Neurodegenerative Disease Research Brain Bank at the University of Pennsylvania. Consent for autopsy was obtained from legal representatives for all subjects in accordance with local institutional review board requirements. In brief, fresh tissues from each brain were fixed with 70% ethanol in 150 mM NaCl, infiltrated with paraffin and cut into 6-μm serial sections. Immunohistochemistry (IHC) was performed using the avidin-biotin complex (ABC) detection system (Vector Laboratories, Burlingame, CA) and 3,3′-diaminobenzidine. In brief, sections were deparaffinized and rehydrated, antigen retrieval was done by incubating section in 88% formic acid, endogenous peroxidases were quenched with 5% H 2 O 2 in methanol for 30 min and sections were blocked in 0.1 mol l −1 Tris with 2% fetal bovine serum for 5 min. Primary antibodies were incubated for either 1 or 2 h at room temperature or overnight at 4 °C. The following primary antibodies were used for IHC analysis: AcK145 (this study, 1:500), monoclonal TDP-43 (Proteintech, 1:1,000), P-409/410 (1:500). After washing, sections were sequentially incubated with biotinylated secondary antibodies for 1 h and avidin–biotin complex for 1 h. Bound antibody complexes were visualized by incubating sections in a solution containing 100 mM TrisHCl, pH 7.6, 0.1% Triton X-100, 1.4 mM diaminobenzidine, 10 mM imidazole and 8.8 mM H 2 O 2 . Sections were then lightly counterstained with haematoxylin, dehydrated and coverslipped. We note that IHC analysis of human tissue using Ac-K145 requires antigen retrieval (formic acid) for maximal detection sensitivity of TDP-43 inclusions and displays mild cross-reactivity with other nuclear proteins. Double-labelling Immunofluorescence - Double-labelling immunofluorescence (IF) analyses were performed using Alexa Fluor 488- and 594-conjugated secondary antibodies (Molecular Probes, Eugene, OR). The sections were then treated to remove autofluorescence with Sudan Black solution for 5 min and coverslipped with Vectashield mounting medium (Vector Laboratories). Digital images were obtained using an Olympus BX 51 microscope (Tokyo, Japan) equipped with bright-field and fluorescence light sources using a ProgRes C14 digital camera (Jenoptik AG, Jena, Germany) and Adobe Photoshop, version 9.0 (Adobe Systems, San Jose, CA) or digital camera DP71 (Olympus) and DP manager (Olympus). How to cite this article : Cohen, T. J. et al . An acetylation switch controls TDP-43 function and aggregation propensity. Nat. Commun. 6:5845 doi: 10.1038/ncomms6845 (2015).